Inflammation driven by tumour-specific Th1 cells protects against B-cell cancer The immune system can both promote and suppress cancer. Chronic inflammation and proinflammatory cytokines such as interleukin (IL)-1 and IL-6 are considered to be tumour promoting. In contrast, the exact nature of protective antitumour immunity remains obscure. Here, we quantify locally secreted cytokines during primary immune responses against myeloma and B-cell lymphoma in mice. Strikingly, successful cancer immunosurveillance mediated by tumour-specific CD4 + T cells is consistently associated with elevated local levels of both proinflammatory (IL-1α, IL-1β and IL-6) and T helper 1 (Th1)-associated cytokines (interferon-γ (IFN-γ), IL-2 and IL-12). Cancer eradication is achieved by a collaboration between tumour-specific Th1 cells and tumour-infiltrating, antigen-presenting macrophages. Th1 cells induce secretion of IL-1β and IL-6 by macrophages. Th1-derived IFN-γ is shown to render macrophages directly cytotoxic to cancer cells, and to induce macrophages to secrete the angiostatic chemokines CXCL9/MIG and CXCL10/IP-10. Thus, inflammation, when driven by tumour-specific Th1 cells, may prevent rather than promote cancer. The immune system can protect against cancer [1] . Elevated numbers of intratumoral T cells predict long-term survival for patients with advanced ovarian carcinoma and colorectal cancer [2] , [3] . Yet, little is known about the exact nature of protective antitumour immune responses. On the other hand, it is well established that chronic inflammation predisposes to cancer. Proinflammatory cytokines such as interleukin (IL)-1 and IL-6 are considered to be essential for tumour progression, and anti-inflammatory drugs have been suggested to treat cancer [4] , [5] , [6] , [7] , [8] , [9] . However, anti-inflammatory treatments may potentially suppress protective antitumour immunity. Strategies to fight malignancies should be based on stimulating rather than suppressing the ongoing immune response against cancer. Therefore, it is crucial to better understand the interplay between immune cells, inflammation and cancer. Tumour-specific CD4 + T cells orchestrate the immune response against cancer. CD4 + T cells are required for cytokine-mediated activation of tumour-specific cytotoxic CD8 + T cells, but they can also eliminate cancer in the absence of CD8 + T cells [10] , [11] . A recent study of patients with breast cancer concluded that high numbers of CD4 + T cells in lymph nodes (LNs) predict disease-free survival [12] . In lung and liver cancer, high CD4:CD8 T-cell ratios were associated with good prognosis [13] , [14] . However, CD4 + T cells may also suppress antitumour immunity [15] . To clarify the mechanism of cancer prevention by CD4 + T cells, we have used idiotype (Id)-specific T-cell receptor transgenic (TCR-TG) mice, which were made homozygous for the severe combined immunodeficiency (SCID) mutation to prevent rearrangement of endogenous TCR chains [11] . In these mice, tumour-specific CD4 + T cells recognize an Id peptide from the variable region of the immunoglobulin light chain of the MOPC315 myeloma, presented on major histocompatibility complex (MHC) class II molecules [16] . Id-specific TCR-TG SCID mice are resistant against subcutaneous (s.c.) inoculation with syngeneic MOPC315 myeloma cells or with Id-transfected F9 B-lymphoma cells, whereas non-transgenic mice develop fatal tumours. Protection is Id-specific, CD4 + T cell-mediated, and does not require the presence of B cells and CD8 + T cells [11] , [17] . To study the mechanisms of cancer rejection by Id-specific TCR-TG mice, we have developed a strategy consisting of embedding injected tumour cells in a collagen gel (Matrigel). The Matrigel functions as an extracellular matrix in which infiltrating immune cells can be analysed at various time points after injection. Using this method, we have reported the first characterization of a successful primary antitumour immune response initiated by naïve CD4 + T cells [18] . In brief, we could show that s.c. injected MOPC315 myeloma cells were surrounded within 3 days by macrophages, which captured tumour-specific antigens. Within 6 days, naïve Id-specific CD4 + T cells became activated in draining LN and subsequently migrated to the incipient tumour site. On recognition of tumour-derived Id peptides presented on MHC class II molecules by macrophages, Id-specific CD4 + T cells were shown to secrete interferon-γ (IFN-γ). Matrigel-infiltrating macrophages became activated by T cell-derived IFN-γ, and could kill MHC class II-negative myeloma cells directly [18] . However, in this previous report the exact function of IFN-γ was not fully defined and the involvement of other cytokines was not investigated. In this study, we have further developed the Matrigel assay to quantify locally secreted cytokines during primary antitumour immune responses. Using this method, we uncovered a common core of nine cytokines that were consistently associated with successful cancer immunosurveillance. Strikingly, this core includes both proinflammatory (IL-1α, IL-1β and IL-6) and T helper (Th)1-associated (IL-2, IL-3, IL-12, IFN-γ, CXCL9 and CXCL10) cytokines. Twelve additional cytokines were associated with cancer prevention in most, but not all experimental settings investigated. Thus, we have identified a total of 21 cytokines, which may serve as a basis to develop cytokine-based immunotherapy for cancer. Furthermore, we provide evidence for a dual antitumour role of Th1-derived IFN-γ. First, IFN-γ triggers tumouricidal activity of tumour-infiltrating macrophages. Second, IFN-γ induces macrophages to secrete the angiostatic chemokines CXCL9/MIG (monokine induced by IFN-γ) and CXCL10/IP-10 (IFN-γ inducible protein 10), which may halt tumour progression by inhibiting angiogenesis. Collectively, our data suggest a cancer-protective role of inflammation driven by tumour-specific Th1 cells. The Matrigel cytokine assay We have developed a method to quantify locally secreted cytokines during the early stages of an immune response against cancer in mice. The method is based on s.c. inoculation of cancer cells embedded in a Matrigel collagen gel ( Fig. 1a ). Matrigel is derived from a murine sarcoma and therefore represents a genuine tumour cell microenvironment [19] . Matrigel, which is liquid at +4 °C, gelifies at body temperature and forms a gel plug containing the injected cancer cells [18] . The gel functions as an extracellular matrix and contains the cytokines that are secreted locally by cancer cells and by infiltrating immune cells. At various time points after injection, the Matrigel plug can be excised and dissolved in vitro with collagenase. A cell-free supernatant containing secreted cytokines that are present in the Matrigel extracellular matrix is obtained by centrifugation ( Fig. 1a ). Cytokines in the supernatant are quantified by multiplex bead assays. An initial experiment to test the method revealed that numerous cytokines could be detected in the Matrigel at day +8, which represents the height of the antitumour immune response [18] ( Supplementary Fig. S1 ). To identify cytokines associated with successful cancer immunosurveillance, we designed a series of five experimental situations to compare cytokine levels during successful versus failed immune responses against cancer. 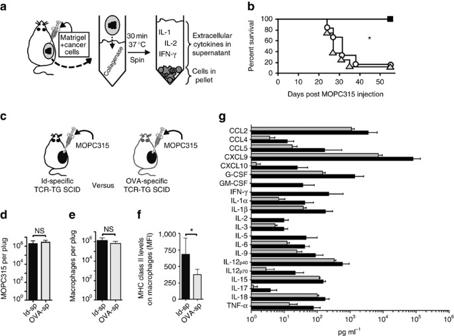Figure 1: Role of tumour-specific CD4+T cells for myeloma immunosurveillance. (a) The Matrigel cytokine assay. Cancer cells are mixed with cold liquid Matrigel before s.c. injection. Matrigel gelifiesin vivoand forms a gel plug. The plug contains the injected cancer cells, infiltrating immune cells and cytokines that are secreted locally. At various time points after injection, the Matrigel plug is excised and dissolved with collagenase. Following centrifugation, cytokines in supernatant are quantified by Luminex technology. Cells in the pellet are analysed by various techniques such as flow cytometry, Luminex technology and gene expression microarrays. (b) Tumour challenge experiment. Id-specific TCR-TG SCID mice (squares), OVA-specific TCR-TG SCID mice (triangles) and SCID mice (circles) were injected s.c. with MOPC315 myeloma cells in phosphate-buffered saline (PBS). Tumour development and survival were followed over time. *P=0.0004 for difference in survival between Id-specific and OVA-specific TCR-TG SCID mice (log-rank test). (c) Design of the first experimental situation for cytokine analysis (myeloma±specific T cells). Id-specific TCR-TG SCID mice and OVA-specific TCR-TG SCID mice were injected s.c. with MOPC315 myeloma cells in Matrigel. The plugs were analysed individually at day +8. (d) Total number of MOPC315 cells per plug. (e) Total number of CD11b+macrophages per plug. (f) MHC class II levels on Matrigel-infiltrating CD11b+macrophages. MFI, mean fluorescence intensity. *P=0.009, Mann–Whitney test. (g) The concentration of 33 cytokines in the extracellular matrix of the Matrigel plugs was quantified for Id-specific (black bars) and OVA-specific (grey bars) TCR-TG SCID mice. Only cytokines with significantly (P<0.05, Mann–Whitney test) higher levels in one group compared with the other are included in the bar graph. (b)n=6–8. (c–g)n=11. Id-sp, Id-specific TCR-TG SCID mice; NS, not significant; OVA-sp, OVA-specific TCR-TG SCID mice. All data are presented as mean±s.d. G-CSF, granulocyte colony-stimulating factor; GM-CSF, granulocyte-macrophage colony-stimulating factor; TNF-α, tumor necrosis factor α. Figure 1: Role of tumour-specific CD4 + T cells for myeloma immunosurveillance. ( a ) The Matrigel cytokine assay. Cancer cells are mixed with cold liquid Matrigel before s.c. injection. Matrigel gelifies in vivo and forms a gel plug. The plug contains the injected cancer cells, infiltrating immune cells and cytokines that are secreted locally. At various time points after injection, the Matrigel plug is excised and dissolved with collagenase. Following centrifugation, cytokines in supernatant are quantified by Luminex technology. Cells in the pellet are analysed by various techniques such as flow cytometry, Luminex technology and gene expression microarrays. ( b ) Tumour challenge experiment. Id-specific TCR-TG SCID mice (squares), OVA-specific TCR-TG SCID mice (triangles) and SCID mice (circles) were injected s.c. with MOPC315 myeloma cells in phosphate-buffered saline (PBS). Tumour development and survival were followed over time. * P =0.0004 for difference in survival between Id-specific and OVA-specific TCR-TG SCID mice (log-rank test). ( c ) Design of the first experimental situation for cytokine analysis (myeloma±specific T cells). Id-specific TCR-TG SCID mice and OVA-specific TCR-TG SCID mice were injected s.c. with MOPC315 myeloma cells in Matrigel. The plugs were analysed individually at day +8. ( d ) Total number of MOPC315 cells per plug. ( e ) Total number of CD11b + macrophages per plug. ( f ) MHC class II levels on Matrigel-infiltrating CD11b + macrophages. MFI, mean fluorescence intensity. * P =0.009, Mann–Whitney test. ( g ) The concentration of 33 cytokines in the extracellular matrix of the Matrigel plugs was quantified for Id-specific (black bars) and OVA-specific (grey bars) TCR-TG SCID mice. Only cytokines with significantly ( P <0.05, Mann–Whitney test) higher levels in one group compared with the other are included in the bar graph. ( b ) n =6–8. ( c – g ) n =11. Id-sp, Id-specific TCR-TG SCID mice; NS, not significant; OVA-sp, OVA-specific TCR-TG SCID mice. All data are presented as mean±s.d. G-CSF, granulocyte colony-stimulating factor; GM-CSF, granulocyte-macrophage colony-stimulating factor; TNF-α, tumor necrosis factor α. Full size image Tumour-specific CD4 + T cells control local cytokine levels In the first experimental situation (myeloma±specific T cells), we compared tumour-specific CD4 + T cells with CD4 + T cells that recognized an irrelevant antigen, ovalbumin (OVA). Id-specific TCR-TG SCID mice, OVA-specific TCR-TG SCID mice and SCID mice were injected s.c. with MOPC315 myeloma cells. Id-specific TCR-TG SCID mice were protected against MOPC315 ( Fig. 1b ), as previously reported [11] . Control SCID mice, which lack T and B cells, succumbed from cancer within 40 days. OVA-specific TCR-TG SCID mice, which have T cells but cannot recognize Id, developed tumours as quickly as SCID mice ( Fig. 1b ). For a cytokine assay, Id-specific and OVA-specific TCR-TG SCID mice were injected with MOPC315 in Matrigel ( Fig. 1c–g ). The total numbers of MOPC315 cells and CD11b + macrophages in Matrigel at day +8 were similar for both groups ( Fig. 1d,e ). However, when we used MHC class II upregulation as an activation marker for macrophages [18] , activated MHC class II high macrophages were only found in Id-specific TCR-TG SCID mice ( Fig. 1f ). Quantification of 33 cytokines in Matrigel revealed that the local concentration of 21 cytokines was significantly higher in the presence of tumour-specific CD4 + T cells, that is, in tumour-resistant Id-specific TCR-TG SCID mice ( Fig. 1g ; Supplementary Fig. S2 ). Notably, cytokine levels in serum were similar between the groups, underscoring the importance of measuring cytokines locally at the incipient tumour site ( Supplementary Fig. S2 ). Cytokines associated with myeloma immunosurveillance We then investigated the role of tumour-specific antigen using an antigen-loss (Ag-loss) variant of MOPC315 which is not rejected by Id-specific TCR-TG SCID mice [20] . In the second experimental situation (myeloma±antigen, one flank), two groups of Id-specific TCR-TG SCID mice were injected with Matrigel containing either MOPC315 or Ag-loss MOPC315 ( Fig. 2a,b ). Matrigel cytokine quantification at day +8 revealed that the local concentration of 21 cytokines was significantly higher when cancer immunity was successful, that is, in mice injected with antigen-producing myeloma cells ( Fig. 2b ; Supplementary Fig. S3 ). In the third experimental situation (myeloma±antigen, two flanks), we designed a system in which successful and failed immunosurveillance could be investigated in the same mouse at different anatomic locations. Id-specific TCR-TG SCID or SCID mice were injected with MOPC315 in Matrigel on the right flank and with Ag-loss MOPC315 in Matrigel on the left flank. SCID mice developed tumours with similar kinetics on both flanks. In contrast, Id-specific TCR-TG SCID mice efficiently suppressed the growth of MOPC315, but failed to reject Ag-loss MOPC315 on the contralateral flank, demonstrating the antigen specificity of the antitumour immune response within the same mouse ( Fig. 2c ). For a Matrigel cytokine assay, Id-specific TCR-TG SCID mice were injected on both flanks with either MOPC315 or Ag-loss MOPC315 ( Fig. 2d–g ). At day +8, activated CD69 + tumour-specific CD4 + T cells were observed in the right-flank LN draining the MOPC315 injection site, but not in the contralateral LN draining Ag-loss MOPC315 ( Fig. 2e ). Activated, MHC class II high macrophages were only detected in the right-flank Matrigel plugs containing MOPC315, but not in the contralateral site ( Fig. 2f ), confirming the importance of antigen presentation in situ for T cell-mediated activation of macrophages [18] . Multiplex bead analysis revealed that local antigen recognition by tumour-specific CD4 + T cells resulted in increased levels of 13 cytokines and decreased levels of 3 cytokines in Matrigel ( Fig. 2g ; Supplementary Fig. S4 ). Analysis of all the MOPC315 data revealed that 11 cytokines were consistently associated with successful immunosurveillance against myeloma ( Table 1 ). 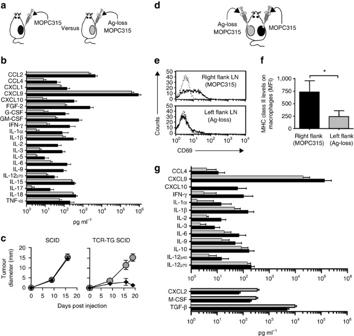Figure 2: Role of antigen for myeloma immunosurveillance. (a) Design of the second experimental situation for cytokine analysis (myeloma±antigen, 1 flank). Id-specific TCR-TG SCID mice were injected s.c. with MOPC315 or with Ag-loss MOPC315 in Matrigel. At day +8, the concentration of 33 cytokines in the extracellular matrix of the Matrigel plugs was quantified for each mouse. (b) Matrigel cytokine levels for mice inoculated with MOPC315 (black bars) or with Ag-loss MOPC315 (grey bars) from the experiment described ina. Only cytokines with significantly (P<0.05) higher levels in one group compared with the other are included in the bar graph. (c) Double-flank tumour challenge experiment. Id-specific TCR-TG SCID or SCID mice were injected with MOPC315 in Matrigel on the right flank (black diamonds), and with Ag-loss MOPC315 in Matrigel on the left flank (grey circles). Tumour development on each side was followed over time. (d) Design of the third experimental situation for cytokine analysis (myeloma±antigen, 2 flanks). Id-specific TCR-TG SCID mice were injected with MOPC315 on the right flank, and with Ag-loss MOPC315 on the left flank. Matrigel plugs and draining LNs were analysed at day +8. (e) Expression of CD69 on gated tumour-specific (GB113+), CD4+T cells in the LN draining the right and left flank from a representative mouse. Dotted lines indicate an isotype-matched control monoclonal antibodies (mAb). (f) MHC class II levels on gated CD11b+macrophages that had infiltrated the Matrigel plugs containing either MOPC315 (right flank) or Ag-loss MOPC315 (left flank). *P=0.0002. (g) Cytokines levels in Matrigel plugs containing either MOPC315 (black bars) or Ag-loss MOPC315 (grey bars). Only cytokines with significantly higher (top) or lower (bottom) levels (P<0.05) in one group compared with the other are included in the graphs. (a,b)n=6. (c)n=7–8. (d–g)n=11. All data are presented as mean±s.d. Statistical analysis was performed with the Mann–Whitney test. FGF-2, fibroblast growth factor 2; M-CSF, macrophage colony-stimulating factor; TGF-β, transforming growth factor-β. Figure 2: Role of antigen for myeloma immunosurveillance. ( a ) Design of the second experimental situation for cytokine analysis (myeloma±antigen, 1 flank). Id-specific TCR-TG SCID mice were injected s.c. with MOPC315 or with Ag-loss MOPC315 in Matrigel. At day +8, the concentration of 33 cytokines in the extracellular matrix of the Matrigel plugs was quantified for each mouse. ( b ) Matrigel cytokine levels for mice inoculated with MOPC315 (black bars) or with Ag-loss MOPC315 (grey bars) from the experiment described in a . Only cytokines with significantly ( P <0.05) higher levels in one group compared with the other are included in the bar graph. ( c ) Double-flank tumour challenge experiment. Id-specific TCR-TG SCID or SCID mice were injected with MOPC315 in Matrigel on the right flank (black diamonds), and with Ag-loss MOPC315 in Matrigel on the left flank (grey circles). Tumour development on each side was followed over time. ( d ) Design of the third experimental situation for cytokine analysis (myeloma±antigen, 2 flanks). Id-specific TCR-TG SCID mice were injected with MOPC315 on the right flank, and with Ag-loss MOPC315 on the left flank. Matrigel plugs and draining LNs were analysed at day +8. ( e ) Expression of CD69 on gated tumour-specific (GB113 + ), CD4 + T cells in the LN draining the right and left flank from a representative mouse. Dotted lines indicate an isotype-matched control monoclonal antibodies (mAb). ( f ) MHC class II levels on gated CD11b + macrophages that had infiltrated the Matrigel plugs containing either MOPC315 (right flank) or Ag-loss MOPC315 (left flank). * P =0.0002. ( g ) Cytokines levels in Matrigel plugs containing either MOPC315 (black bars) or Ag-loss MOPC315 (grey bars). Only cytokines with significantly higher (top) or lower (bottom) levels ( P <0.05) in one group compared with the other are included in the graphs. ( a , b ) n =6. ( c ) n =7–8. ( d – g ) n =11. All data are presented as mean±s.d. Statistical analysis was performed with the Mann–Whitney test. FGF-2, fibroblast growth factor 2; M-CSF, macrophage colony-stimulating factor; TGF-β, transforming growth factor-β. Full size image Table 1 Cytokine profiles of successful cancer immunosurveillance. * Full size table Cytokines consistently associated with cancer prevention To assess the general significance of our findings, we performed an experiment with another cancer type, namely the F9 B-cell lymphoma. F9 is an A20 BALB/c-derived lymphoma that was transfected with Id, whereas F55 is an Id-negative control lymphoma [21] . As F9 but not F55 cells are rejected by Id-specific TCR-TG mice [17] , this model represents successful versus failed immunosurveillance against lymphoma. An important difference between the two cancer types is that MOPC315 cells do not express MHC class II molecules, whereas F9 cells express high levels and thus can present Id directly to CD4 + T cells [21] . Id-specific TCR-TG SCID mice were injected with F9 cells in Matrigel on the right flank, and with F55 cells in Matrigel on the left flank. In addition, SCID mice were injected with F9 cells in Matrigel ( Fig. 3a–c ). Activated, MHC class II high macrophages were only detected in Matrigel containing Id-expressing F9 in TCR-TG SCID mice, but not in Matrigel with F55, nor in SCID mice ( Fig. 3b ). Thus, the activation of Matrigel-infiltrating macrophages required (i) the presence of Id-specific CD4 + T cells and (ii) the local production of Id antigen. This observation suggests that the antitumour immune response may be very similar against MOPC315 and F9 cells, although the two cell types differ in terms of MHC class II expression. Cytokine quantification of all Matrigel plugs allowed two separate analyses of the data. First, cytokine levels were compared between each flank of the TCR-TG SCID mice (lymphoma±antigen, two flanks). The local levels of 19 cytokines were higher in right-flank Matrigel plugs containing F9, compared with left-flank Matrigel plugs containing F55 ( Fig. 3c ; Supplementary Fig. S5 ). In a second parallel analysis of the data (lymphoma±specific T cells), Matrigel plugs containing F9 were compared between TCR-TG SCID and SCID mice, revealing increased levels of 20 cytokines in the situation in which immunosurveillance against lymphoma was successful, that is, in Id-specific TCR-TG mice ( Table 1 ; Supplementary Fig. S5 ). Analysis of all the F9 data showed that 16 cytokines were consistently associated with successful immunosurveillance against B-cell lymphoma ( Table 1 ). Further analysis revealed a common core of nine cytokines that were consistently associated with successful cancer immunosurveillance against myeloma and lymphoma: IL-1α, IL-1β, IL-2, IL-3, IL-6, IL-12p70, IFN-γ, CXCL9 and CXCL10 ( Table 1 ). Twelve additional cytokines were associated with cancer rejection in most but not all situations investigated ( Table 1 ). 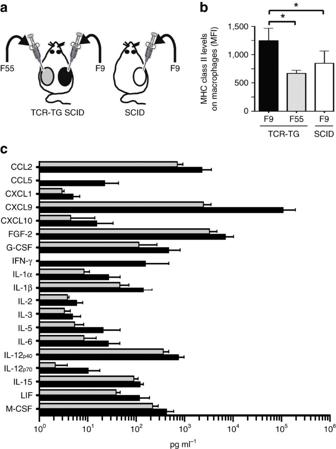Figure 3: Immunosurveillance of B-cell lymphoma. (a) Design of the fourth (lymphoma±antigen, 2 flanks) and fifth (lymphoma±specific T cells) experimental situations for cytokine analysis. Id-specific TCR-TG SCID mice were injected s.c. with Id+F9 B-lymphoma cells in Matrigel on the right flank, and with Id−F55 B-lymphoma cells in Matrigel on the left flank. SCID mice were injected s.c. with Id+F9 cells in Matrigel on the right flank. Matrigel plugs were analysed at day +8. (b) Expression of MHC class II on gated CD11b+macrophages that had infiltrated the Matrigel plugs for each group of samples. (c) Cytokines in Matrigel were quantified. Data for Id+F9 (black bars) versus Id−F55 (grey bars) in TCR-TG SCID mice are shown in the bar graph for cytokines with significantly (P<0.05) higher levels in one group compared with the other. (a–c)n=10–11. *P<0.001. All data are presented as mean±s.d. Statistical analysis was performed with the Mann–Whitney test. Figure 3: Immunosurveillance of B-cell lymphoma. ( a ) Design of the fourth (lymphoma±antigen, 2 flanks) and fifth (lymphoma±specific T cells) experimental situations for cytokine analysis. Id-specific TCR-TG SCID mice were injected s.c. with Id + F9 B-lymphoma cells in Matrigel on the right flank, and with Id − F55 B-lymphoma cells in Matrigel on the left flank. SCID mice were injected s.c. with Id + F9 cells in Matrigel on the right flank. Matrigel plugs were analysed at day +8. ( b ) Expression of MHC class II on gated CD11b + macrophages that had infiltrated the Matrigel plugs for each group of samples. ( c ) Cytokines in Matrigel were quantified. Data for Id + F9 (black bars) versus Id − F55 (grey bars) in TCR-TG SCID mice are shown in the bar graph for cytokines with significantly ( P <0.05) higher levels in one group compared with the other. ( a – c ) n =10–11. * P <0.001. All data are presented as mean±s.d. Statistical analysis was performed with the Mann–Whitney test. Full size image Role of IFN-γ IFN-γ-deficient (IFN-γ −/− ) Id-specific TCR-TG SCID mice were unable to reject MOPC315 or F9 cells, demonstrating the critical role of IFN-γ for immunosurveillance of both myeloma and lymphoma ( Fig. 4a ). Interestingly, tumour growth was significantly delayed in IFN-γ −/− Id-specific TCR-TG SCID mice as compared with SCID mice, suggesting residual, but insufficient antitumour immunity in the absence of IFN-γ ( Fig. 4a ). For a Matrigel cytokine assay, IFN-γ +/+ and IFN-γ −/− Id-specific TCR-TG SCID mice were injected with MOPC315 ( Fig. 4b–f ). At day +8, activated CD69 + Id-specific T cells were found for both groups of mice in draining LNs and in Matrigel plugs ( Fig. 4c ). Thus, IFN-γ was required neither for activation of naïve tumour-specific T cells in LNs nor for their migration and reactivation at the incipient tumour site. In fact, significantly more tumour-specific T cells were found in the Matrigel plugs from IFN-γ −/− mice ( Fig. 4d ), presumably because T-cell proliferation is generally stronger in IFN-γ −/− mice [22] . Although activated Matrigel-infiltrating tumour-specific T cells were present in both groups, activated MHC class II high macrophages were only detected in the plugs from IFN-γ +/+ mice ( Fig. 4e ), confirming the importance of IFN-γ for macrophage activation [18] . Matrigel cytokine quantification revealed that the local levels of three cytokines (IFN-γ, CXCL9 and CXCL10) were significantly lower, whereas one cytokine (IL-1β) was higher, in IFN-γ −/− compared with IFN-γ +/+ mice ( Fig. 4f ; Supplementary Fig. S6 ). Thus, IFN-γ deficiency results in reduced secretion of CXCL9 and CXCL10 at the incipient tumour site. 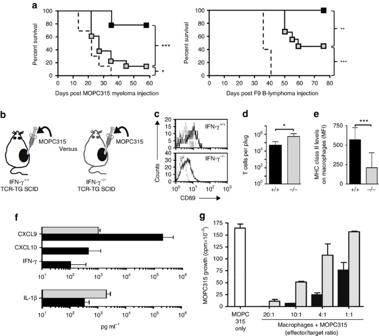Figure 4: Role of IFN-γ for tumour protection and local cytokine production. (a) Tumour challenge experiments. IFN-γ+/+Id-specific TCR-TG SCID mice (black squares), IFN-γ−/−Id-specific TCR-TG SCID mice (grey squares) and IFN-γ+/+SCID mice (dotted line) were injected s.c. with MOPC315 myeloma cells (left panel) or with F9 B-lymphoma cells (right panel) in PBS. Tumour development and survival were followed over time by palpation. (b) Experimental design for Matrigel cytokine assay. Id-specific TCR-TG SCID IFN-γ+/+and IFN-γ−/−mice were injected s.c. with MOPC315 in Matrigel. At day +8, Matrigel-infiltrating T cells and macrophages were analysed, and locally secreted cytokines were quantified. (c) Expression of CD69 on Matrigel-infiltrating, tumour-specific T cells (GB113+TCRCβ+) from representative IFN-γ+/+and IFN-γ−/−mice. Dotted lines indicate an isotype-matched control mAb. (d) Total number of tumour-specific T cells (GB113+TCRCβ+) per plug for IFN-γ+/+and IFN-γ−/−mice. (e) Expression of MHC class II on gated CD11b+macrophages that had infiltrated the Matrigel plugs in IFN-γ+/+and IFN-γ−/−mice. (f) The concentration of 33 cytokines in Matrigel was quantified. Only cytokines with significantly higher (top) or lower (bottom) levels (P<0.05) in IFN-γ+/+(black bars) mice compared with IFN-γ−/−(grey bars) mice are included in the bar graphs. (g) Growth inhibition assay. Id-specific TCR-TG SCID IFN-γ+/+and IFN-γ−/−mice were injected s.c. with Matrigel containing MOPC315. Matrigel-infiltrating CD11b+macrophages were purified at day +7 and tested at various effector to target ratios for their ability to suppress the proliferation of MOPC315 cellsin vitro. Black bars, macrophages from IFN-γ+/+mice; grey bars, macrophages from IFN-γ−/−mice. (a)n=5–14. (b–f)n=11. (g) triplicates. *P<0.05, **P<0.01, ***P<0.001. Statistical analysis was performed with the log-rank test (a) and the Mann–Whitney test (d–f). All data are presented as mean±s.d. Figure 4: Role of IFN-γ for tumour protection and local cytokine production. ( a ) Tumour challenge experiments. IFN-γ +/+ Id-specific TCR-TG SCID mice (black squares), IFN-γ −/− Id-specific TCR-TG SCID mice (grey squares) and IFN-γ +/+ SCID mice (dotted line) were injected s.c. with MOPC315 myeloma cells (left panel) or with F9 B-lymphoma cells (right panel) in PBS. Tumour development and survival were followed over time by palpation. ( b ) Experimental design for Matrigel cytokine assay. Id-specific TCR-TG SCID IFN-γ +/+ and IFN-γ −/− mice were injected s.c. with MOPC315 in Matrigel. At day +8, Matrigel-infiltrating T cells and macrophages were analysed, and locally secreted cytokines were quantified. ( c ) Expression of CD69 on Matrigel-infiltrating, tumour-specific T cells (GB113 + TCRCβ + ) from representative IFN-γ +/+ and IFN-γ −/− mice. Dotted lines indicate an isotype-matched control mAb. ( d ) Total number of tumour-specific T cells (GB113 + TCRCβ + ) per plug for IFN-γ +/+ and IFN-γ −/− mice. ( e ) Expression of MHC class II on gated CD11b + macrophages that had infiltrated the Matrigel plugs in IFN-γ +/+ and IFN-γ −/− mice. ( f ) The concentration of 33 cytokines in Matrigel was quantified. Only cytokines with significantly higher (top) or lower (bottom) levels ( P <0.05) in IFN-γ +/+ (black bars) mice compared with IFN-γ −/− (grey bars) mice are included in the bar graphs. ( g ) Growth inhibition assay. Id-specific TCR-TG SCID IFN-γ +/+ and IFN-γ −/− mice were injected s.c. with Matrigel containing MOPC315. Matrigel-infiltrating CD11b + macrophages were purified at day +7 and tested at various effector to target ratios for their ability to suppress the proliferation of MOPC315 cells in vitro . Black bars, macrophages from IFN-γ +/+ mice; grey bars, macrophages from IFN-γ −/− mice. ( a ) n =5–14. ( b – f ) n =11. ( g ) triplicates. * P <0.05, ** P <0.01, *** P <0.001. Statistical analysis was performed with the log-rank test ( a ) and the Mann–Whitney test ( d – f ). All data are presented as mean±s.d. Full size image In a previous report, we have shown that Matrigel-infiltrating macrophages, isolated from Id-specific TCR-TG SCID mice, were cytotoxic to MOPC315 cells in vitro [18] . Tumouricidal macrophage activity was strictly dependent on macrophage activation by CD4 + T cells, because macrophages isolated from SCID mice, even in high numbers, could not inhibit MOPC315 growth. It was speculated that macrophages were rendered tumouricidal by Th1-derived IFN-γ [18] . To test this hypothesis, we compared the tumouricidal activity of macrophages isolated from either IFN-γ +/+ or IFN-γ −/− TCR-TG SCID mice. The ability of Matrigel-infiltrating macrophages from IFN-γ −/− mice to inhibit the growth of MOPC315 cells in vitro was severely reduced, although not completely abolished ( Fig. 4g ). Hence, IFN-γ is required for rendering tumour-infiltrating macrophages fully competent to directly kill cancer cells. Myeloma immunosurveillance is mediated by Th1 cells IFN-γ is a typical product of activated Th1 cells but tumour-specific Th17 cells may also secrete IFN-γ [23] . Intracellular flow cytometry revealed that Matrigel-infiltrating Id-specific T cells produced IFN-γ and tumour necrosis factor α (TNF-α), and expressed the transcription factor T-bet, which is consistent with a Th1 differentiation. In contrast, Id-specific T cells did not express molecular markers for Th2 (IL-4, Gata-3), Th17 (IL-17) or regulatory T cells (Foxp3; Fig. 5a ). Thus, myeloma rejection in Id-specific TCR-TG SCID mice is mediated by IFN-γ-producing tumour-specific Th1 cells. 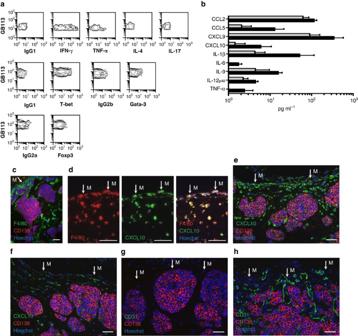Figure 5: Cytokine production of tumour-specific CD4+T cells and macrophages. (a) Characterization of Matrigel-infiltrating tumour-specific T cells by intracellular flow cytometry. Id-specific TCR-TG SCID mice (n=12–15) were injected s.c. with MOPC315 in Matrigel. At day +8, Matrigel plugs were excised and pooled. Matrigel-infiltrating tumour-specific (GB113+TCRCβ+) T cells were stained for intracellular cytokines and for transcription factors. IgG1, IgG2a and IgG2b indicate isotype-matched control mAb. (b) Measurement of intracellular cytokines in Matrigel-infiltrating macrophages. Id-specific TCR-TG SCID mice or SCID mice (n=12–15) were injected with MOPC315 in Matrigel. At day +8, Matrigel-infiltrating CD11b+macrophages were purified and pooled for groups of 3–4 mice. Sorted macrophages were washed and lysed. Cytokines in cell lysates were quantified by Luminex technology. The bar graph represents cytokine levels in macrophages from Id-specific TCR-TG SCID mice (black bars) and from SCID mice (grey bars) for cytokines with significantly (P<0.05, Mann–Whitney test) higher levels in one group compared with the other (mean±s.d.). For the purpose of comparison, cytokine levels were corrected to 2×105macrophages per pool. (c) Visualization of successful myeloma immunosurveillance. MOPC315 myeloma cells were injected in Matrigel into a tumour-resistant Id-specific TCR-TG SCID mouse. At day +8, a tissue sample containing the Matrigel plug was excised for immunohistochemistry. Matrigel-infiltrating macrophages were stained with anti-F4/80 (green) mAb. MOPC315 myeloma cells were stained with anti-CD138 (red) mAb. Hoechst stain (blue) was used to visualize cell nuclei. (d) A day +8, sample from a tumour-resistant Id-specific TCR-TG SCID mouse was double-stained with F4/80 (red) and CXCL10 (green). (e) CXCL10 (green) production by Matrigel-infiltrating macrophages in a tumour-resistant Id-specific TCR-TG SCID mouse. MOPC315 myeloma cells were stained with anti-CD138 mAb (red). (f) CXCL10 (green) production by Matrigel-infiltrating macrophages in a tumour-prone OVA-specific TCR-TG SCID mouse. (g) Anti-CD31 polyclonal antibodies were used to stain blood vessels in a tumour-resistant Id-specific TCR-TG SCID mouse. (h) Formation of CD31+(green) blood vessels around CD138+(red) myeloma tumour islets in a tumour-prone SCID mouse. Immunostaining images (c–h) show representative day +8 specimens for groups of ≥3 mice. Scale bars, 50 μm. M, edge of Matrigel plug. Figure 5: Cytokine production of tumour-specific CD4 + T cells and macrophages. ( a ) Characterization of Matrigel-infiltrating tumour-specific T cells by intracellular flow cytometry. Id-specific TCR-TG SCID mice ( n =12–15) were injected s.c. with MOPC315 in Matrigel. At day +8, Matrigel plugs were excised and pooled. Matrigel-infiltrating tumour-specific (GB113 + TCRCβ + ) T cells were stained for intracellular cytokines and for transcription factors. IgG1, IgG2a and IgG2b indicate isotype-matched control mAb. ( b ) Measurement of intracellular cytokines in Matrigel-infiltrating macrophages. Id-specific TCR-TG SCID mice or SCID mice ( n =12–15) were injected with MOPC315 in Matrigel. At day +8, Matrigel-infiltrating CD11b + macrophages were purified and pooled for groups of 3–4 mice. Sorted macrophages were washed and lysed. Cytokines in cell lysates were quantified by Luminex technology. The bar graph represents cytokine levels in macrophages from Id-specific TCR-TG SCID mice (black bars) and from SCID mice (grey bars) for cytokines with significantly ( P <0.05, Mann–Whitney test) higher levels in one group compared with the other (mean±s.d.). For the purpose of comparison, cytokine levels were corrected to 2×10 5 macrophages per pool. ( c ) Visualization of successful myeloma immunosurveillance. MOPC315 myeloma cells were injected in Matrigel into a tumour-resistant Id-specific TCR-TG SCID mouse. At day +8, a tissue sample containing the Matrigel plug was excised for immunohistochemistry. Matrigel-infiltrating macrophages were stained with anti-F4/80 (green) mAb. MOPC315 myeloma cells were stained with anti-CD138 (red) mAb. Hoechst stain (blue) was used to visualize cell nuclei. ( d ) A day +8, sample from a tumour-resistant Id-specific TCR-TG SCID mouse was double-stained with F4/80 (red) and CXCL10 (green). ( e ) CXCL10 (green) production by Matrigel-infiltrating macrophages in a tumour-resistant Id-specific TCR-TG SCID mouse. MOPC315 myeloma cells were stained with anti-CD138 mAb (red). ( f ) CXCL10 (green) production by Matrigel-infiltrating macrophages in a tumour-prone OVA-specific TCR-TG SCID mouse. ( g ) Anti-CD31 polyclonal antibodies were used to stain blood vessels in a tumour-resistant Id-specific TCR-TG SCID mouse. ( h ) Formation of CD31 + (green) blood vessels around CD138 + (red) myeloma tumour islets in a tumour-prone SCID mouse. Immunostaining images ( c – h ) show representative day +8 specimens for groups of ≥3 mice. Scale bars, 50 μm. M, edge of Matrigel plug. Full size image Cytokine production of tumouricidal macrophages We then quantified intracellular cytokines in sorted populations of Matrigel-infiltrating macrophages. Macrophages involved in tumour rejection were purified from Id-specific TCR-TG SCID mice injected with MOPC315, whereas control macrophages were from SCID mice. Successful antitumour immunity was associated with elevated levels of nine cytokines in Matrigel-infiltrating macrophages ( Fig. 5b ; Supplementary Fig. S7 ). These data suggest that, among the cytokines consistently associated with successful cancer immunosurveillance, CXCL9, CXCL10, IL-1β and IL-6, were produced by macrophages on activation by tumour-specific CD4 + T cells. Two additional cytokines (IL-1α and IL-12p70) are also likely to be macrophage-derived because they were present in macrophages, although their levels were not significantly different between TCR-TG SCID and SCID mice ( Supplementary Fig. S7 ). The three remaining cytokines in the common core (IL-2, IL-3 and IFN-γ) are typical T-cell products, and therefore most likely secreted by Matrigel-infiltrating Id-specific Th1 cells. Production of CXCL10 by macrophages was further investigated by immunohistochemistry. CXCL10 was detected in F4/80 + macrophages that penetrated the Matrigel plugs containing CD138 + MOPC315 cells ( Fig. 5c,d ). Matrigel-infiltrating macrophages produced more CXCL10 in tumour-resistant Id-specific TCR-TG SCID mice as compared with tumour-prone OVA-specific mice ( Fig. 5e,f ). Strikingly, successful myeloma immunosurveillance in Id-specific TCR-TG SCID mice was characterized by the absence of angiogenesis, whereas formation of CD31 + blood vessels around tumour islets was readily observable in control mice ( Fig. 5g,h ). This suggests that IFN-γ-activated macrophages use simultaneously two strategies to fight cancer: direct killing of cancer cells ( Fig. 4g ) and indirect inhibition of tumour growth through secretion of angiostatic chemokines such as CXCL9 and CXCL10 ( Fig. 5b–h ). Myeloma immunosurveillance is an inflammatory reaction Histological analysis revealed that myeloma rejection by Id-specific TCR-TG SCID mice was characterized by local inflammation with oedema and inflammatory cell infiltrate ( Fig. 6a ). Matrigel-infiltrating macrophages were further characterized by gene expression microarrays ( Fig. 6b ) and flow cytometry ( Fig. 6c ). Tumouricidal macrophages were isolated from Id-specific TCR-TG SCID mice injected with MOPC315-containing Matrigel. Control macrophages were obtained from TCR-TG SCID mice injected with Matrigel containing Ag-loss MOPC315. The expression of CXCL9 and CXCL10 was upregulated in tumouricidal macrophages compared with controls, confirming that these angiostatic chemokines were produced by T cell-activated macrophages ( Fig. 6b , left panel). Interestingly, several other chemokines were upregulated, including CXCL11/I-TAC (interferon-inducible T-cell α chemokine), another IFN-γ-inducible angiostatic chemokine, CCL17/TARC (thymus and activation regulated chemokine) and CCL22/MDC (macrophage-derived chemokine). The levels of CCL17 and CCL22 in Matrigel samples from the myeloma experiments were measured by enzyme-linked immunosorbent assay, but no association with successful immunosurveillance was found ( Supplementary Fig. S8 ). Tumouricidal macrophages showed upregulation of genes associated with antigen processing and presentation ( Fig. 6b , right panel), and increased levels of MHC class II and co-stimulatory molecules such as CD40, CD80, CD86, CD273 and CD274 ( Fig. 6c ). Hence, tumouricidal macrophages have a typical phenotype of activated professional antigen-presenting cells. 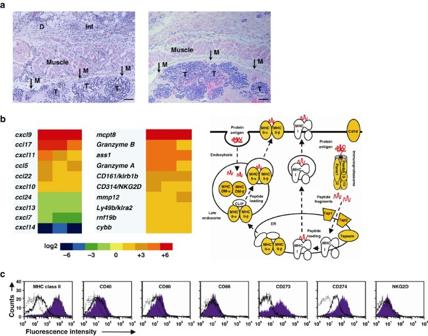Figure 6: Myeloma immunosurveillance is an inflammatory reaction. (a) Tumour-resistant Id-specific and tumour-prone OVA-specific TCR-TG SCID mice were injected s.c. with MOPC315 myeloma cells in Matrigel. Tissue samples were taken at day +8 and sections were stained with hematoxylin and eosin. Successful myeloma immunosurveillance in an Id-specific TCR-TG SCID mouse is characterized by inflammation with oedema and infiltration of inflammatory cells (left panel). Such inflammatory features are not observed in a control OVA-specific TCR-TG SCID mouse (right panel). Representative images for groups of ≥3 mice are shown. Scale bars, 100 μm. D, dermis; Inf, inflammatory cell infiltrate; M, edge of Matrigel plug; T, tumour cell islet. (b) Gene expression was compared for tumouricidal/control macrophages. Matrigel-infiltrating, tumouricidal macrophages were isolated at day +8 from Id-specific TCR-TG SCID mice (n=12–15) injected with MOPC315-containing Matrigel. Control macrophages were obtained from Id-specific TCR-TG SCID mice (n=12–15) injected with Matrigel containing Ag-loss MOPC315. The expression of all known genes was quantified by gene microarrays. Data for chemokines (left panel) and cytotoxicity-associated genes (middle panel) that were differentially expressed are shown. Each column indicates one independent experiment. The cartoon (right panel) illustrates the antigen processing and presentation pathway. Proteins encoded by genes whose expression was consistently ≥2 times higher in tumouricidal macrophages in three independent experiments are shown in yellow.ass1, argininosuccinate synthetase 1;cybb, cytochrome b-245 beta polypeptide; ER, endoplasmic reticulum;mcpt8, mast cell protease 8;mmp12, matrix metalloproteinase 12; Psm, proteasome subunit;rnf19b, ring finger protein 19B; Tap, transporter associated with antigen processing. (c) Characterization of Matrigel-infiltrating macrophages at day +8 by flow cytometry. Gated Matrigel-infiltrating CD11b+cells were analysed in Id-specific TCR-TG SCID mice injected s.c. with either MOPC315 (shaded blue area) or Ag-loss MOPC315 (boldface line). Dotted lines indicate isotype-matched control mAb. Multiple experiments were conducted with similar results. Figure 6: Myeloma immunosurveillance is an inflammatory reaction. ( a ) Tumour-resistant Id-specific and tumour-prone OVA-specific TCR-TG SCID mice were injected s.c. with MOPC315 myeloma cells in Matrigel. Tissue samples were taken at day +8 and sections were stained with hematoxylin and eosin. Successful myeloma immunosurveillance in an Id-specific TCR-TG SCID mouse is characterized by inflammation with oedema and infiltration of inflammatory cells (left panel). Such inflammatory features are not observed in a control OVA-specific TCR-TG SCID mouse (right panel). Representative images for groups of ≥3 mice are shown. Scale bars, 100 μm. D, dermis; Inf, inflammatory cell infiltrate; M, edge of Matrigel plug; T, tumour cell islet. ( b ) Gene expression was compared for tumouricidal/control macrophages. Matrigel-infiltrating, tumouricidal macrophages were isolated at day +8 from Id-specific TCR-TG SCID mice ( n =12–15) injected with MOPC315-containing Matrigel. Control macrophages were obtained from Id-specific TCR-TG SCID mice ( n =12–15) injected with Matrigel containing Ag-loss MOPC315. The expression of all known genes was quantified by gene microarrays. Data for chemokines (left panel) and cytotoxicity-associated genes (middle panel) that were differentially expressed are shown. Each column indicates one independent experiment. The cartoon (right panel) illustrates the antigen processing and presentation pathway. Proteins encoded by genes whose expression was consistently ≥2 times higher in tumouricidal macrophages in three independent experiments are shown in yellow. ass1 , argininosuccinate synthetase 1; cybb , cytochrome b-245 beta polypeptide; ER, endoplasmic reticulum; mcpt8 , mast cell protease 8; mmp12 , matrix metalloproteinase 12; Psm, proteasome subunit; rnf19b , ring finger protein 19B; Tap, transporter associated with antigen processing. ( c ) Characterization of Matrigel-infiltrating macrophages at day +8 by flow cytometry. Gated Matrigel-infiltrating CD11b + cells were analysed in Id-specific TCR-TG SCID mice injected s.c. with either MOPC315 (shaded blue area) or Ag-loss MOPC315 (boldface line). Dotted lines indicate isotype-matched control mAb. Multiple experiments were conducted with similar results. Full size image Gene expression analysis revealed a number of cytotoxicity-associated genes, which were upregulated in tumouricidal macrophages and which may be involved in the direct killing of cancer cells: proteases ( mcpt8, mmp12 ); granzyme A and B; ass1 and cybb (involved in nitric oxide and superoxide production, respectively); and several genes known to be expressed by natural killer (NK) cells (CD161/ klrb1b , CD314/NKG2D, Ly49b/ klra2 and rnf19b ; Fig. 6b , middle panel; Supplementary Data S1 and S2 ). Moderate upregulation of NKG2D was confirmed at protein level ( Fig. 6c ). The presence of NK-associated genes in the microarray data is unlikely to originate from cell contamination because we could not detect Matrigel-infiltrating NKp46 hi NK cells by flow cytometry. Furthermore, we performed an experiment with beige mutant mice with a functional defect in NK-cell lytic functions [24] . Id-specific TCR-TG SCID beige mice were fully protected against challenge with MOPC315, indicating that NK cells were not involved in myeloma rejection ( Supplementary Fig. S9 ). Bioinformatic analysis of the upregulated genes in tumouricidal macrophages showed highly significant overlaps with genes or proteins known to be induced in macrophages by IFN-γ ( Supplementary Data S3 ). Furthermore, promoter region analysis revealed that the upregulated genes were enriched for binding sites for inflammation-associated transcription factors such as nuclear factor-κB and RelA ( Supplementary Data S3 ). Thus, myeloma immunosurveillance is an inflammatory reaction characterized by tissue infiltration by IFN-γ-activated macrophages with a typical inflammatory phenotype. We have developed a method to quantify locally secreted cytokines during primary antitumour immune responses in mice. Using this method, we have identified a common core of nine cytokines consistently associated with successful cancer eradication: IL-1α, IL-1β, IL-2, IL-3, IL-6, IL-12p70, IFN-γ, CXCL9 and CXCL10. To our knowledge, these data represent the first characterization of the cytokine profile of successful cancer immunosurveillance. Interestingly, in patients with hepatocellular carcinoma, increased expression of 17 genes in the liver, including IL-1α, IL-1β, IL-2, IL-12 and IFN-γ, was associated with good prognosis [25] . Thus, the cytokine profile of protective immunity against cancer may be very similar for mice and humans. The observation that IL-12 and IFN-γ were constantly associated with cancer rejection is consistent with a Th1 polarization of the immune response, which is widely considered to be favourable for immunological control of cancer [1] , [2] , [3] , [26] . In contrast, the presence in the list of the proinflammatory cytokines IL-1α, IL-1β and IL-6 may seem more surprising. Chronic inflammation predisposes to cancer and cancer-related inflammation is generally regarded as being tumour promoting [4] , [5] , [6] , [7] , [8] , [9] . Elevated IL-1β levels were associated with shorter survival and disease progression in patients with chronic myelogenous leukaemia and colorectal carcinoma [5] , [27] . In mice, IL-1 was shown to be required for tumour invasiveness and angiogenesis [4] , [28] . In several human malignancies, including multiple myeloma, lymphoma and lung cancer, high serum levels of IL-6 were associated with poor prognosis [29] , [30] , [31] . Furthermore, IL-6 was shown to be required for obesity-induced tumour promotion in a mouse model for hepatocellular carcinoma [9] . Although inflammation is generally considered to be tumour promoting, a few histopathological studies in colorectal, breast and bladder cancer indicated that tumour infiltration by inflammatory cells may be associated with better prognosis [32] , [33] , [34] . To reconcile these opposing views, we propose that inflammation, when driven by tumour-specific Th1 cells, may prevent cancer ( Fig. 7a ). In a Th1 environment, proinflammatory cytokines (IL-1α, IL-1β and IL-6) may participate in cancer eradication by recruiting leucocytes from the circulation and by stimulating CD4 + T-cell functions [35] , [36] . In contrast, other types of inflammation, or inflammation that lacks tumour specificity, may not protect and may even promote tumour development ( Fig. 7b ). Hence, caution should be taken when considering anti-inflammatory treatments against cancer [4] , [5] , [6] , [7] . Drugs that may dampen the tumour-suppressive Th1-driven inflammatory immune response should preferably be avoided. 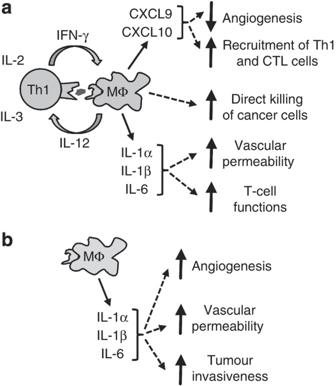Figure 7: A model for how inflammation may either suppress or promote cancer. (a) Tumour-suppressive inflammation. Successful cancer immunosurveillance is mediated by a tumour-specific Th1-driven inflammation. In this process, tumour-specific Th1 cells collaborate with tumour-infiltrating macrophages, and nine cytokines synergize to prevent cancer. Proinflammatory cytokines (IL-1α, IL-1β and IL-6) participate in tumour eradication by recruiting immune cells from the circulation and by stimulating T-cell functions. (b) Tumour-promoting inflammation. In the absence of sufficient numbers of tumour-specific Th1 cells, IL-1α, IL-1β and IL-6 may participate in tumour progression by stimulating angiogenesis, vascular permeability and tumour invasiveness. MΦ, macrophage; CTL, cytotoxic CD8+T cells. Figure 7: A model for how inflammation may either suppress or promote cancer. ( a ) Tumour-suppressive inflammation. Successful cancer immunosurveillance is mediated by a tumour-specific Th1-driven inflammation. In this process, tumour-specific Th1 cells collaborate with tumour-infiltrating macrophages, and nine cytokines synergize to prevent cancer. Proinflammatory cytokines (IL-1α, IL-1β and IL-6) participate in tumour eradication by recruiting immune cells from the circulation and by stimulating T-cell functions. ( b ) Tumour-promoting inflammation. In the absence of sufficient numbers of tumour-specific Th1 cells, IL-1α, IL-1β and IL-6 may participate in tumour progression by stimulating angiogenesis, vascular permeability and tumour invasiveness. MΦ, macrophage; CTL, cytotoxic CD8 + T cells. Full size image The finding that elevated levels of IL-1 (α and β) were consistently associated with successful cancer immunosurveillance is of particular interest. IL-1 is a canonical proinflammatory cytokine, which exerts a broad range of activities including activation of vascular endothelium, stimulation of lymphocyte functions, induction of acute-phase response and fever. The IL-1 receptor and the Toll-like receptors share a common intracellular signalling pathway, which leads to activation of the nuclear factor-κB and to the transcription of several proinflammatory cytokines, including IL-1 itself. Thus, IL-1 functions as a positive feedback loop in inflammation. IL-1 was shown to enhance the expansion and differentiation of CD4 + T cells [35] , [36] , and to induce macrophage tumouricidal activity in vitro [37] . Importantly, IL-1β secretion by macrophages is dependent on activation of the inflammasome, a cytosolic molecular complex responsible for generating active IL-1β by cleaving the inactive precursor. The inflammasome functions as a guardian of the body by detecting pathogens and danger [38] . In cancer immunosurveillance, the nature of the endogenous danger signals detected by the inflammasome remains to be determined, but a role for ATP released by necrotic tumour cells has been suggested [39] . The importance of IFN-γ for cancer immunosurveillance is well documented [1] , [40] , [41] , but its exact function remains poorly understood. IFN-γ was originally defined as a cytokine able to render macrophages tumouricidal in vitro [42] . However, the in vivo relevance of this finding remained unclear. Our data with IFN-γ-deficient mice provide direct evidence for a role of IFN-γ in inducing macrophage tumouricidal activity in vivo . Furthermore, we demonstrate another function of IFN-γ, namely induction of secretion of MIG/CXCL9 and IP-10/CXCL10 by tumour-infiltrating macrophages. CXCL10 selectively attracts Th1 cells [43] and may thus function as a positive feedback loop in the Th1-driven antitumour immune response. Th1-induced CXCL9 and CXCL10 may also be important for recruiting CD8 + T cells to the incipient tumour site [44] . Moreover, neovascularization is required for a solid tumour to grow [45] . Several endogenous angiostatic factors have been described including CXCL9 and CXCL10, which both binds to the CXCR3-B receptor on endothelial cells, resulting in suppression of endothelial cell proliferation and differentiation into capillary structures [46] , [47] , [48] . Treatment with recombinant CXCL9 and CXCL10 was shown to delay tumour growth in mice by inducing vascular damage and tumour necrosis [49] , [50] , [51] . It has been previously suggested that tumour-specific CD4 + T cells may mediate tumour rejection by inhibiting angiogenesis through secretion of IFN-γ [41] , but the mechanism remained obscure. Our results provide direct evidence that IFN-γ, secreted locally by tumour-specific Th1 cells, induces tumour-infiltrating macrophages to secrete the angiostatic chemokines CXCL9 and CXCL10. Since the discovery of the antitumour properties of TNF-α in 1975 (ref. 52 ), there has been a considerable interest in using cytokines to treat patients with cancer. Significant benefits have been demonstrated in the treatment of various malignancies with TNF-α, IL-2 and IFN-α [53] , [54] , [55] , [56] . Other candidate molecules such as granulocyte-macrophage colony-stimulating factor, IL-7, IL-12p70 and IL-15 have shown promising antitumour effects [57] , [58] . However, only a few cytokines are being routinely used to treat cancer. A major challenge to develop cytokine-based immunotherapy is that cytokine networks are based on synergistic interactions [59] . Therefore, coadministration of different cytokines is likely to be required to efficiently treat cancer, as suggested by experiments with mice [59] , [60] . With more than 200 different cytokines described to date, the number of combinations to be tested for cancer therapy is enormous. Our study identified 9 cytokines that were consistently associated with successful antitumour immunity, and 12 additional cytokines that were associated with cancer eradication in most but not all situations investigated. This list should be helpful for the development of combined cytokine-based immunotherapy for cancer. Mice, cell lines and injection of tumour cells Heterozygous Id-specific TCR-TG SCID mice or SCID littermates were on BALB/c background [11] . IFN-γ −/− BALB/c mice [22] (from The Jackson Laboratory) were crossed with Id-specific TCR-TG SCID mice to obtain IFN-γ −/− Id-specific TCR-TG SCID mice. OVA-specific TCR-TG SCID mice were generated by introducing the scid mutation into DO11.10 TCR-TG mice (from Taconic). MOPC315 (IgA, λ2 315 ) is a transplantable BALB/c plasmacytoma obtained from the American Type Culture Collection (ATCC) and propagated as in vitro growing cells. Ag-loss MOPC315.36 (ref. 20 ) was kindly provided by Alexander Marks, University of Toronto. F9 is an A20 BALB/c-derived B-lymphoma cell line that was transfected with Id-containing λ2 315 (ref. 21 ). F55 is an Id-negative lymphoma obtained by transfecting A20 cells with pSV2neo vector without insert [21] . Adult mice were injected s.c., in the interscapular region or in the flank, with 1–1.6×10 5 cancer cells suspended either in 100 μl phosphate-buffered saline (PBS, Gibco), or in 250 μl Growth Factor-Reduced Matrigel (BD Biosciences). Tumour growth was followed over time by palpation. Mice with tumour a diameter ≥10 mm were killed. The study was approved by the National Committee for Animal Experiments (Oslo, Norway). Matrigel cytokine assay Cancer cells were mixed with ice-cold Matrigel and 250 μl of the mixture was carefully injected s.c. into each mouse under anaesthesia. Matrigel, which is liquid at +4 °C, gelifies at body temperature and forms a gel plug containing the injected cancer cells. At day +8, mice were sacrificed. The s.c. Matrigel plug was excised and treated with 1 ml RPMI 1640 medium (Gibco) supplemented with 1 mg ml −1 collagenase type IV from Clostridium histolyticum and 0.3 mg ml −1 DNase I from bovine pancreas (Sigma), at 37 °C for 30 min. Dissolved Matrigel solution was squeezed through a stainless steel sieve (Sigma) and centrifuged 300 g for 7 min. The cell pellet was analysed by flow cytometry. Cell-free supernatant was pressed through a 0.45 μm syringe filter (PALL Corporation) and kept at −70 °C until analysis by Luminex technology. To test the method, tumour-resistant Id-specific TCR-TG SCID mice were injected s.c. with either Matrigel containing MOPC315 cells or with empty Matrigel, as a control. At day +8, the Matrigel plugs were excised for cytokine analysis. For comparison, a Matrigel solution was used to generate in vitro plugs, which were processed similarly. The concentration of 33 cytokines in the extracellular matrix of the Matrigel plugs was quantified by Luminex technology. This experiment showed that the Matrigel solution itself ( in vitro or ex vivo ) only contains very low levels of cytokines, except for transforming growth factor-β and vascular endothelial growth factor, which were high. In contrast, numerous cytokines were detected in the day +8 MOPC315-containing Matrigel plugs recovered from s.c. injections ( Supplementary Fig. S1 ). Preparation of macrophage lysates TCR-TG SCID mice ( n =12) or SCID mice ( n =14) were injected s.c. with 10 5 MOPC315 cells in 250 μl Matrigel. At day +8, Matrigel-infiltrating CD11b + macrophages were sorted by FACSAria (≥ 95% pure) and pooled for groups of three to four mice. Sorted macrophages (1.5–3×10 5 per pool) were washed and lysed in a buffer containing 5 mM EDTA, 50 mM Tris-HCL pH7.0, 0.5% NP-40 and 150 mM NaCl (all from Sigma). Lysates were pressed through a 0.45 μm syringe filter and kept at −70 °C until analysis by Luminex technology. Cytokine quantification by Luminex technology Cytokine levels in Matrigel supernatants, cell lysates and serum were measured using single-plex or multiplex bead assays from Bio-Rad Laboratories (Bio-Plex 23-plex and 9-plex panels) and Biosource Invitrogen (for TGF-β and CXCL-10), according to the manufacturer's instructions. Samples were analysed as singlets and standards in duplicates, using a Luminex-100 instrument with Bio-Plex Manager 4.1 software (Bio-Rad Laboratories). Analysis of cells by flow cytometry Single-cell suspension from draining axillary LNs and Matrigel plugs were obtained by use of a stainless steel sieve. Unspecific binding was blocked by incubation with heat-inactivated (56 °C, 30 min) 30% normal rat serum in PBS and 100 μg ml −1 anti-FcγRII/III monoclonal antibodies (mAb; clone 2.4G2). Cells were stained for 15 min on ice with specific mAbs in PBS supplemented with 0.5% bovine serum albumin (Biotest). The following commercially available mAbs were used, conjugated with either fluorescein, phycoerythrin, allophycocyanin or biotin: CD4 (RM4.5 or GK1.5), CD11b (M1/70), CD273 (TY25), CD274 (MIH5), CD314 (CX5), IFN-γ (XMG1.2), IL-4 (11B11), IL-17 (TC11-18H10), MHC class II I-A/I-E (M5/114.15.2), TCRCβ (H57-597), TNF-α (MP6-XT22) (BD Biosciences); CD11b (3A33), CD40 (1C10), CD69 (H1.2F3), CD80 (1G10), CD86 (GL1) (Southern Biotechnology); Foxp3 (FJK-16s), Gata-3 (TWAJ), T-bet (4B10) (eBioscience). The following mAbs were affinity-purified and, if needed, biotinylated in our laboratory: anti-Id-specific-TCR-clonotype (GB113), anti-FcγRII/III (2.4G2; ATCC). Biotinylated mAbs were detected with streptavidin conjugated to peridinin chlorophyll protein (BD Biosciences). For intracellular cytokine detection, cells were stimulated with phorbol myristate acetate and ionomycin (both from Sigma) in vitro for 4 h in cell culture medium supplemented with monensin, before staining with Cytofix/Cytoperm Plus reagents (BD Biosciences) and specific mAbs. Quadruple-stained cells were analysed on a FACSCalibur instrument with CellquestPro software (BD Biosciences). Tumour cell growth inhibition assay Matrigel-infiltrating CD11b + cells were purified by FACSAria at day +7 after s.c. injection. Sorted CD11b + cells (≥95% pure) were irradiated (2,000 rad) and added at various effector/target ratios to MOPC315 cell cultures (10 4 tumour cells per well) in triplicates. Cultures were pulsed with [ 3 H]thymidine after 48 h and collected 12 h later on a TopCount NXT microplate counter. Tissue preparation The Matrigel plugs were removed by a wide excision of the flank wall, including the skin. Tissue samples were either flash frozen in O.C.T. compound (Tissue-Tek) in liquid nitrogen and stored at −80 °C, or fixed in 10% buffered formaldehyde and paraffin-embedded. Four micrometre tissue sections were cut from the tissue blocks. Frozen sections were air-dried overnight and subsequently acetone-fixed. Paraffin-embedded sections were deparaffinized with xylene, and bathed consecutively in absolute ethanol, 96% ethanol, 70% ethanol and PBS. Sections for light microscopy were stained with hematoxylin for 3 min, hexamine for 3 min and eosin for 45 s, and subsequently dehydrated with xylene. Immunohistochemistry The paired immunostainings for F4/80+CD138 and F4/80+CXCL10 were performed on frozen sections, whereas the other stainings were done on formalin-fixed paraffin-embedded tissue sections. Frozen tissue sections were incubated with the primary and secondary antibodies for 1 h each at room temperature. To visualize CXCL10, we amplified the signal by means of a secondary antibody horseradish peroxidase-conjugated goat anti-rabbit IgG and Alexa 488-conjugated tyramide amplification reagent according to manufacturer's instructions (Invitrogen). For paraffin-embedded sections, antigen retrieval was performed on deparaffinized, formalin-fixed tissue sections by boiling those for 20 min in 10 mM Tris-EDTA pH 9. Sections were then incubated with the primary antibodies overnight at 4 °C, followed by the secondary antibodies for 1 h at room temperature. Hoechst blue nuclear stain was added to the final volume of washing buffer after the last incubation. As negative controls, primary irrelevant isotype- and concentration-matched antibodies were used. Samples were examined with a Nikon Eclipse E-800 fluorescence microscope (Nikon) equipped with Nikon Plan-Fluor objective lenses and an F-VIEW digital camera controlled by AnalySIS 3.2 software (Soft Imaging System GmbH). Antibodies and all working concentrations are listed in Supplementary Tables S1 and S2 . Gene expression analysis Id-specific TCR-TG SCID mice were injected s.c. with Matrigel containing 10 5 MOPC315 cells. At day +8, Matrigel-infiltrating CD11b + tumouricical macrophages were sorted by FACSAria (≥95% pure) in three independent experiments. Control macrophages were obtained similarly in two independent experiments from Id-specific TCR-TG SCID mice injected with Matrigel containing Ag-loss MOPC315 cells. TRIzol (Invitrogen) was used to extract mRNA from sorted macrophages. The expression of all known genes was quantified by gene microarrays (GeneChip Mouse Genome 430 2.0 Array, Affymetrix). Changes in gene expression (≥2) that were consistent for all sample comparisons (tumouricidal/control macrophages) were considered to be significant. The microarray expression data sets were deposited in Gene Expression Omnibus (GEO, www.ncbi.nlm.nih.gov/geo ) under accession number GSE26912 . Statistical analysis For tumour challenge experiments, differences in survival were analysed with the log-rank test. Flow cytometry data and cytokine levels were analysed with the Mann–Whitney test. Statistical analysis was performed with GraphPad Prism 4 software. Accession codes: Expression data sets were deposited in GEO under accession number GSE26912 . How to cite this article: Haabeth, O.A.W. et al . Inflammation driven by tumour-specific Th1 cells protects against B-cell cancer. Nat. Commun. 2:240 doi: 10.1038/ncomms1239 (2011).